Foxgspecifies sensory neurons in the anterior neural plate border of the ascidian embryo Foxg constitutes a regulatory loop with Fgf8 and plays an important role in the development of anterior placodes and the telencephalon in vertebrate embryos. Ascidians, which belong to Tunicata, the sister group of vertebrates, develop a primitive placode-like structure at the anterior boundary of the neural plate, but lack a clear counterpart of the telencephalon. In this animal, Foxg is expressed in larval palps, which are adhesive organs with sensory neurons. Here, we show that Foxg begins to be expressed in two separate rows of cells within the neural plate boundary region under the control of the MAPK pathway to pattern this region. However, Foxg is not expressed in the brain, and we find no evidence that knockdown of Foxg affects brain formation. Our data suggest that recruitment of Fgf to the downstream of Foxg might have been a critical evolutionary event for the telencephalon in the vertebrate lineage. Although the brain of ascidians, which belong to the sister group of vertebrates, is much simpler than the vertebrate brain, it is organized with several regionalized structures. Indeed, the posterior part of the ascidian brain is regionalized by Fgf8 [1] , which is reminiscent of the vertebrate midbrain-hindbrain boundary organizer [2] , [3] . However, ascidians lack a clear counterpart of the telencephalon, the most anterior part of the vertebrate central nervous system. The anterior ectodermal ridge, from which cranial placodes are derived, is required for the formation of the telencephalon in vertebrate embryos [4] , [5] . Vertebrate cranial placodes are now considered to share their evolutionary origin with the anterior boundary region of the neural plate of ascidian embryos [6] , [7] , [8] , [9] , [10] , [11] , [12] . Therefore, the anterior boundary region of the neural plate of the ascidian embryo may lack the inducing activity to regionalize the anterior part of the brain. Foxg is a transcription factor important for development of the telencephalon and cranial placodes in vertebrate embryos [13] , [14] . In ascidian embryos, Foxg is expressed in palps [12] , [15] , which are adhesive organs with sensory neurons [16] , [17] , [18] . This region is derived from the abovementioned anterior neural plate border regions (ANB), which is located in the anterior border between the neural plate and epidermal cells [7] , [11] , [15] , [18] . In the present study, we examined how Foxg is used for formation of the ANB cells in the ascidian embryo to eventually understand the evolution of the placodes and the telencephalon. In ascidian embryos, specification of the ANB begins with expression of Foxc at the gastrula stage [7] , [8] . The four cells expressing Foxc delineate the anterior border of the neural plate and divide twice along the anterior–posterior axis until the neurula stage (Fig. 1a ). Among the resultant four rows of cells, the most posterior row expresses Six1/2 and contributes to the oral siphon primordium, which is formed in the region anterior to the brain and contains sensory neurons [11] . The anterior three rows of cells mainly contribute to the palps. Three cell types are readily recognizable in the palps of Ciona larvae by three molecular markers [18] , although there may be more cell types in this region [16] . Cells with Isl expression have an elongated shape and are found in the palp protrusions, while cells with Emx expression surround the cells expressing Isl at the base of the protrusions. Zf220 , which encodes a protein related to vertebrate Sp6/Sp7/Sp8/Sp9 transcription factors, is expressed in anterior ectodermal cells intervening among the three palps as well as in the cells with Emx expression [18] . Fig. 1 Foxg is specifically expressed in two rows of the anterior border of the neural plate. a Schematic illustrations of the anterior border of the neural plate in ascidian embryos. Epidermal cells, neural plate cells, and the intervening cells are represented by white, cyan, and yellow rectangles, respectively. b – d Foxg expression revealed by chromatic and fluorescence in situ hybridization at the early and late neurula stages. Foxg is initially expressed in two separate rows during the neurula stage, and cells in the anterior row divide along the mediolateral axis until the late neurula stage. e – i Double fluorescence in situ hybridization showing expression of e Foxg (green) and Six1/2 (magenta), f Foxg (green) and Emx (magenta), g , h Foxg (green) and Zf220 (magenta), and i Foxg (green) and Isl (magenta) at the late neurula to middle tailbud stages. Photographs are Z-projected image stacks overlaid in pseudocolor. The brightness and contrast of these photographs were adjusted linearly. Nuclei stained by DAPI are shown in gray in some photographs. j Depictions of the expression patterns of Foxg, Six1/2 , Emx , and Zf220 in the neural plate border at the neurula stage. b , e Dorsal views in which the anterior is up. c , d , f – i Anterior views in which the ventral side is up. Ant anterior, Post posterior, Dor dorsal, Vent ventral. Scale bars represent 50 μm Full size image Here we demonstrate that Foxg plays a key role in establishing these specific expression patterns in the anterior boundary region of the neural plate. More specifically, Foxg begins to be expressed under the control of the MAPK pathway in two separate rows of cells in the boundary region, and regulates Emx , Zf220 , and Isl . However, Foxg is not expressed in the neural plate cells that contribute to the brain, and no apparent effects are observed in the brain of Foxg morphant larvae. Our data suggest a possibility that recruitment of Fgf to the downstream of Foxg had been a critical evolutionary event for the telencephalon in the vertebrate lineage. Foxg is expressed in the anterior neural plate boundary The ANB cells are derived from cells expressing Foxc , which begins to be expressed in one row of cells adjacent to the most anterior cells of the neural plate at the gastrula stage [7] , [15] , [19] (Fig. 1a ). By the early neurula stage, these cells divide twice and produce four rows of cells. In situ hybridization showed that Foxg was expressed in the most anterior and posterior rows of these four rows, but not in the intervening two rows (Fig. 1b, c ). Then, the cells in the anterior row divided in the mediolateral direction and continued to express Foxg (Fig. 1d ; see also Fig. 1j ). To confirm that cells with Foxg expression were ANB-lineage cells, we performed double in situ hybridization of Foxg and Six1/2 at the late neurula stage (Fig. 1e ), because Six1/2 is expressed in eight cells that are derived from cells with and without Foxc expression [11] . Foxg was indeed expressed only in the central four cells derived from cells with Foxc expression. A previous study has shown that Emx begins to be expressed at the neurula stage [18] . In the present study, we determined the precise identities of cells with Emx expression at the neurula stage. At the late neurula stages, Emx was expressed in the middle two rows between the most anterior row and the most posterior row with Foxg expression (Fig. 1f ). At the initial tailbud stage, Foxg expression became weak in the posterior row (Fig. 1g ). Among the eight cells in the anterior row, four cells began to express Zf220 , which is known to be expressed in the palp-forming region [15] , [18] , [19] (Fig. 1g ). The Foxg expression was rarely detectable at the early tailbud stage and became visible again in three spots that form palp protrusions at the middle tailbud stage (Fig. 1h ). At this stage, Foxg and Zf220 were expressed in a mutually exclusive manner (Fig. 1h ). Cells with Foxg expression also expressed Isl (Fig. 1i ), which is expressed in cells with an elongated shape within the palp protrusions and regulates morphogenesis of the palps [18] . The expression patterns of Foxg , Six1/2 , Emx , and Zf220 in the ANB at the early neurula to initial taibud stages are summarized in Fig. 1j . To examine whether Foxg was expressed after metamorphosis, we performed reverse-transcription and PCR (RT-PCR). As shown in Fig. 2a , we detected Foxg expression in neurulae, tailbud embryos, and 5-day juveniles but rarely in mature adults, while we detected control Ef1α expression in all samples. Next, to determine which tissues in juveniles expressed Foxg , we cut a juvenile into four pieces as shown in Fig. 2b . While Ef1α expression was detected in all samples, Foxg expression was detected only in the piece containing cells derived from the palps (specimen 4), but not in the pieces containing the oral siphon, the brain, or the remaining body part (specimens 1 to 3) (Fig. 2c ). Thus, it is not likely that Foxg is expressed in the brain region after metamorphosis. Fig. 2 Foxg is not expressed in the nervous system after metamorphosis. a RT-PCR assay for Foxg expression in neurula embryos, tailbud embryos, juveniles, and adults. Ef1α expression was examined for a positive control. No amplification is observed in the negative control (RT- control), in which water was added instead of reverse transcriptase. b A juvenile in the same age used for RT-PCR in ( a ) and ( c ). For preparation of specimens used in ( c ), we cut animals into four pieces as indicated by lines. These four pieces are called specimens 1 to 4. The scale bar represents 50 μm. c RT-PCR assay for Foxg expression in four pieces of juveniles. Ef1α expression was examined for a positive control. No Foxg expression was detected in specimens 1 to 3 Full size image Foxg is required for palp formation The expression pattern of Foxg implied that it functions in palp formation. We therefore knocked down Foxg by two specific morpholino antisense oligonucleotides (MOs). The first one was designed to block splicing, and the second one was designed to block translation. Injection of either of these MOs resulted in loss of palp protrusions, suggesting that these MOs specifically suppressed Foxg functions (Fig. 3a–c ). In addition, we confirmed that the first MO indeed blocked splicing of nascent Foxg RNA by reverse-transcription followed by PCR (RT-PCR) (Supplementary Fig. 1 ). Specifically, because this MO was designed to bind to the boundary between the second exon and second intron, we prepared PCR primers to amplify fragments containing the entire second and third exons (Supplementary Fig. 1a, b ). While we obtained a single band from control uninjected embryos by RT-PCR, we obtained multiple bands from neurula and tailbud embryos developed from eggs injected with the splice-blocking MO (Supplementary Fig. 1c ). We cloned these PCR products and determined their sequences in 27 randomly picked clones. All of them were different from the expected sequence of the normal transcript (Supplementary Fig. 1d ). These observations indicated that these MOs specifically suppressed Foxg functions, and that Foxg was required for palp formation. Fig. 3 Foxg is essential for palp formation. a – c Morphology of the larval trunk developed from a control unperturbed eggs, b eggs injected with a MO designed to block splicing of Foxg RNA, and c eggs injected with a MO designed to block translation of Foxg mRNA. While two of three palp protrusions are visible in normal embryos shown in ( a ) (arrowheads), no palp protrusions are visible in the morphants shown in ( b ) and ( c ). d , e Isl expression in embryos injected with d the control lacZ mRNA and e the Foxg MO. The palp-forming region lost Isl expression in the Foxg morphant shown in ( e ) (arrowhead). Lateral views are shown. f A larva in which Foxg was over/misexpressed using the upstream region of Foxc developed a single large palp (arrowhead). g , h The ANB cells were marked with GFP by introducing the Foxc > Foxg construct and counterstained with phalloidin (gray). The anterior trunk regions of g a control larva and h a larva in which Foxg was over/misexpressed are shown. g In normal embryos, ANB cells contribute to the palp region and the oral siphon primordium (arrowhead). h In embryos with Foxg over/misexpression, all Gfp-positive cells were found in the single large palp. i , j Isl expression in ( i ) a control embryo and ( j ) an embryo with Foxg over/misexpression. Isl is expressed in the entire palp-forming region in ( j ). k , l Fluorescence in situ hybridization for Emx and Rfp . Embryos were injected with k the lacZ MO or l the Foxg MO. Foxg > Rfp was coinjected to mark the most anterior and posterior rows of the ANB and detected by in situ hybridization. In ( l ), ectopic expression of Emx was detected in the anterior row. The number of embryos examined and the proportion of embryos that each panel represents are shown within the panels. The brightness and contrast of fluorescence images were adjusted linearly. Scale bars represent 50 μm Full size image Concomitantly, Isl was not expressed in the palps of Foxg morphants, while it was expressed normally in embryos injected with the control MO against E. coli lacZ (Fig. 3d, e ). Because over/misexpression of Isl with the Foxc upstream region produces a single large palp [18] , we similarly over/misexpressed Foxg with the same regulatory sequence (the construct was designated as Foxc > Foxg ). Over/misexpression of Foxg led to the formation of a single large palp (Fig. 3f ). We simultaneously introduced Foxc > Gfp to mark cells with Foxc expression. According to the cell lineage, cells with Foxc expression were found in the palps, their intervening region, and the oral siphon primordium of normal embryos (Fig. 3g ). In embryos introduced with Foxc > Foxg , all cells labeled with GFP were found in the large palp, and they had an elongated shape (Fig. 3h ). Specifically, overexpression of Foxg can convert all cells with Foxc expression to palp cells with an elongated shape. Concomitantly, Isl was expressed in all cells in the palp-forming region including the intervening cells at the tailbud stage (Fig. 3i, j ). Thus, Foxg positively regulates Isl expression in the palps. In normal embryos, Foxg and Emx were mutually exclusively expressed in the ANB. Therefore, we examined the possibility that Foxg repressed Emx . For this purpose, we marked the anterior and posterior rows of the ANB by coinjection of Foxg > Rfp with the control lacZ MO or Foxg MO. As shown in Fig. 3k , l, Emx was expressed ectopically in the most anterior row of the ANB of Foxg morphants at the late neurula stage. Thus, Foxg specifies the fate of elongated cells in the palps by activating Isl and repressing Emx . Although the posterior row of the ANB contributes to the oral siphon primordium, no clear morphological changes were observed around the oral siphon primordium in Foxg morphants (Fig. 4a, b ). Concomitantly, Pitx expression in cells anterior to the oral opening [20] , [21] was not changed at the tailbud stage (Fig. 4c, d ), and Six1/2 expression was not changed at the neurula stage (Fig. 4e, f ). The anterior neural ridge, which expresses Foxg , plays an important role in patterning the forebrain of vertebrate embryos [13] , [14] . However, in the ascidian embryo, no clear changes were observed in the morphology or expression of Foxb and Meis , which mark different cells in the anterior part of the brain [22] (Fig. 4g–j ). These observations suggest that Foxg does not function in patterning the anterior part of the brain. Fig. 4 Knockdown of Foxg does not affect the anterior part of the brain. a , b Confocal images of the trunk region of middle tailbud embryos injected with a the lacZ MO or b the Foxg MO, which were stained with phalloidin. Arrowheads indicate the oral opening. Two layers of cells from the oral opening to the middle part of the brain are marked with magenta dots. c – j In situ hybridization of c , d Pitx , e , f Six1/2 , g , h Foxb , and i , j Meis in embryos injected with c , e , g , i the lacZ MO or d , f , h , j the Foxg MO. The number of embryos examined and the proportion of embryos that each panel represents are shown within the panels. Scale bars represent 50 μm Full size image In vertebrates, Foxg is also involved in proper formation of the inner ear, which is derived from the otic placode [23] , [24] . A pair of the atrial siphon primordia has been suggested to be a counterpart of the otic placode [10] , [25] . However, Foxg was not expressed in the atrial siphon primordia or their precursors, as we showed in Fig. 1 . In addition, we did not observe any morphological defects in the atrial siphon primordia in Foxg morphants (Fig. 5 ), suggesting that Foxg is not required for formation of the atrial siphon primordia in ascidian embryos. Fig. 5 Knockdown of Foxg does not affect the atrial siphon primordia. Z-projected images of the trunk region of a a control larva and b a larva developed from an egg injected with the Foxg MO, which were stained with phalloidin. Arrowheads indicates the anterior tip. Note that the palps were lost in the Foxg morphant larva. Atrial siphon primordia in the right side are shown in higher magnification views. The openings are indicated by arrows. In higher magnification views, nuclei are stained by DAPI are shown in gray Full size image Zf220 restricts Foxg expression to three spots of cells As shown in Fig. 1g and h, Zf220 began to be expressed in four cells with Foxg expression at the neurula stage, and then these two genes became expressed in different cells by the middle tailbud stage. Therefore, we tested the hypothesis that Zf220 repressed Foxg . While Foxg was expressed in three spots of cells of control embryos, Foxg was expressed ectopically in embryos injected with a MO to block translation of Zf220 (Fig. 6a, b ); Foxg was expressed ectopically in the intervening cells of the spots, and its expression pattern consequently became an arc shape (Fig. 6b ). Conversely, over/misexpression of Zf220 using the Foxc upstream regulatory sequence resulted in loss of Foxg expression (Fig. 6c ). Although we were not able to obtain another effective MO for Zf220 , it was highly likely that the above effect was specific for the following reasons. First, the morphology of morphants appeared normal at the early to middle tailbud stage, suggesting that the MO did not affect normal development non-specifically. Second, over/misexpression of Zf220 produced the opposite phenotype. Thus, the above results indicated that Zf220 restricted the expression domain of Foxg in a small number of cells that eventually expressed Isl . Fig. 6 Zf220 restricts Foxg expression to cells forming palp protrusions. In situ hybridization of Foxg in tailbud embryos introduced with a the lacZ MO, b the Zf220 MO, and c an over/mis-expression construct of Zf220 ( Foxc > Zf220 ). The number of embryos examined and the proportion of embryos that each panel represents are shown within the panels. The scale bar in ( a ) represents 50 μm Full size image Upstream regulatory factors for Foxg expression A previous study has suggested that Foxg is regulated by Foxc at the tailbud stage [12] . Therefore, we examined whether Foxc also regulated Foxg expression at the neurula stage. As expected, Foxg expression was lost in embryos injected with a Foxc MO (Fig. 7a, b ). Therefore, Foxc is required for the initial expression of Foxg at the neurula stage. Fig. 7 Upstream mechanism that regulates specific expression of Foxg . a – c Foxg expression in embryos injected with a the lacZ control MO, b the Foxc MO, and c the Tfap2-r.b MO. Rows that express Foxg are shown by black arrowheads, and rows that lose the expression are shown by white arrowheads. d Immunostaining of dpERK (magenta) in an embryo in which ANB cells were marked with Foxc > Gfp . The brightness and contrast of fluorescence images were adjusted linearly. Note that dpERK signals are also seen in the most anterior row of the neural plate. e Depiction of dpERK-positive cells in the ANB. f – i In situ hybridization of f , g Foxg and h , i Emx in f , h control embryos and g , i embryos treated with U0126. The number of embryos examined and the proportion of embryos that each panel represents are shown within the panels. The scale bar in ( a ) represents 50 μm Full size image Tfap2 plays an important function in specifying the neural plate border in vertebrate embryos, and it may have played an important role in the evolution of these specific cells [26] , [27] . Although Tfap2-r.b is essential to specify the epidermal fate in Ciona embryos [28] , it had not been determined whether it is required for ANB specification. As shown in Fig. 7c , the expression of Foxg was lost in the anterior row, but not in the posterior row of Tfap2-r.b morphants. This result indicated that Foxg is regulated differently in the anterior and posterior rows, and that Tfap2-r.b is required for Foxg expression in the anterior row. Foxg was expressed only in the anterior and posterior rows of cells of the ANB derived from cells with Foxc expression. Therefore, we next investigated why Foxg was expressed only in two of the four rows. Because the MAPK signaling pathway is repeatedly used in patterning of the nervous system of the ascidian embryo [1] , [29] , [30] , [31] , [32] , [33] , [34] , we examined the possibility that Foxg expression was also regulated by this signaling pathway. Immunostaining with a specific antibody against doubly phosphorylated ERK (dpERK) showed that this signaling pathway was activated in the anterior and posterior rows of the ANB, but not in the middle two rows (Fig. 7d, e ). Treatment with a MEK inhibitor, U0126, indeed resulted in loss of Foxg expression and ectopic Emx expression in the anterior and posterior rows of the ANB (Fig. 7f–i ). These results indicated that the MAPK pathway activated Foxg expression and repressed Emx expression in the anterior and posterior rows of the ANB. Foxg is negatively regulated by ephrin signals Next, we examined why the MAPK signaling pathway was activated only in the anterior and posterior rows of the ANB. Because Ephrina.d ( Efna.d ) is specifically expressed in the ANB at the neurula stage [15] , and because Efna.d is repeatedly used to suppress the activity of the MAPK signaling pathway in ascidian embryos [30] , [33] , [35] , [36] , [37] , we examined the possibility that Efna.d was involved in the specific expression of Foxg and Emx . First, we determined the identities of cells expressing Efna.d . Double in situ hybridization of Efna.d and Foxg revealed that all ANB cells expressed Efna.d (Fig. 8a, b ). Fig. 8 Efna.d is responsible for restricting Foxg expression in the ANB. a Double in situ hybridization of Efna.d (magenta) and Foxg (green). b Depiction for Efna.d expression in the ANB. c Immunostaining of dpERK (magenta) in an embryo in which ANB cells were marked with Foxc > Gfp . The middle rows show ectopic signals for dpERK (arrowheads). d Depiction of ANB cells stained with the anti-dpERK antibody in neurula embryos introduced with Foxc > dn-Eph.c . e – g In situ hybridization of e Foxg and f , g Emx in e , g neurula embryos introduced with Foxc > dn-Eph.c and f an unperturbed neurula embryo. In ( e ), the middle two rows of cells expressed Foxg ectopically (compared with Fig. 1b ). In ( f ) and ( g ), while Emx expression in the tail was not changed, it was lost in the ANB of a Foxg morphant (arrowhead). The number of embryos examined and the proportion of embryos that each panel represents are shown within the panels. a , c , e Anterior views in which the ventral side is up. f , g Dorsal views in which the anterior is up. h Lateral view showing the morphology of a larva introduced with Foxc > dn-Eph.c . ANB cells were marked with GFP by cointroduction of the Foxc > Gfp construct and counterstained with phalloidin (gray) Full size image Second, to confirm that ephrin signaling indeed repressed the MAPK pathway in the anterior and posterior rows of the ANB, we misexpressed a dominant negative form of an ephrin receptor, Eph.c, under the control of the Foxc upstream sequence, because it has been demonstrated that this dominant negative form functions effectively in the ascidian embryo [33] . In embryos introduced with this overexpression construct, dpERK signals were detected in the middle rows of the ANB (Fig. 8c, d ). Therefore, it was likely that the ephrin signaling indeed negatively regulated the MAPK pathway. Concomitantly, Foxg was ectopically expressed in the middle two rows of neurula embryos introduced with the misexpression construct (Fig. 8e ). As a result, Emx expression was abolished in the ANB (Fig. 8f, g ). The resultant larvae had a single large palp as was the case for over/misexpression of Foxg (Fig. 8h ). Thus, the action of Efna.d establishes the specific expression patterns of Foxg and Emx in the ANB by controlling MAPK pathway activity. Foxc is first expressed in the anterior border of the neural plate of the ascidian embryo [7] , [15] . As summarized in Fig. 9 , under the control of this transcription factor, the most anterior and posterior rows of cells expressed Foxg . Because Foxg repressed Emx , Emx is expressed specifically in the intervening two rows. Later, Foxg expression disappeared in the posterior row that gives rise to the oral siphon primordium. Similarly, it disappeared in several cells of the anterior row, because Zf220 negatively regulated Foxg . Zf220 is regulated directly or indirectly by Foxc [19] . Subsequently, Foxg activated Isl , which promotes cell elongation in the palps [18] . Thus, Foxg specified the fate of cells that elongated in the palp. Furthermore, Foxg played a role in restricting Emx expression and thereby indirectly regulated the fate of cells located in the basal region of the palps. Fig. 9 Foxg plays a central role in patterning the ANB. The gene regulatory circuit in the ANB revealed by the present and previous studies [7] , [12] , [18] , [19] Full size image On the other hand, we did not observe any changes in gene expression of the oral siphon primordium. Although we could not rule out the possibility that Foxg has target genes, which we did not assess, in the posterior rows of the ANB, no obvious morphological changes were observed. Therefore, Foxg may not be important for differentiation of this organ. As we mentioned above, Foxg was regulated by Foxc . In addition, it is regulated by the MAPK signaling pathway activated in the most anterior and posterior rows of the ANB, but not in the middle two rows. Efna.d , which is expressed in all four rows derived from cells with Foxc expression, was responsible for this differential activation. Because Efna.d encodes a membrane-anchored signaling ligand that negatively regulates the MAPK pathway, it is expected that the MAPK pathway is suppressed more strongly in the middle two rows of cells than in the anterior and posterior rows of cells. Similar mechanisms have been revealed in earlier embryos [30] , [33] , [35] , [36] , [37] . Specifically, among cells expressing Efna.d , centrally located cells are expected to receive more Efna.d signals, because they are surrounded only by cells expressing Efna.d . On the other hand, marginally located cells are expected to receive less signals, because they are surrounded by cells with and without Efna.d expression. Thus, the MAPK signaling pathway is activated strongly in the anterior and posterior rows among the four rows of the ANB. An unsolved issue is which molecules activate the MAPK pathway. The MAPK signaling pathway is potentially activated in the entire ANB, as revealed in embryos introduced with the dominant negative form of the Eph.c receptor. Therefore, ligand molecules may be expressed in the entire ANB and/or its nearby region. Although Fgf8 induces Foxg expression in vertebrate embryos [4] , its ortholog is unlikely expressed in the ANB of the ascidian embryo [1] , [38] . In addition, it is also unlikely that other genes encoding Fgf molecules are expressed there [38] . Ligands other than Fgf molecules may activate this pathway in the ANB of the ascidian embryo. In vertebrate embryos, Foxg is expressed in the telencephalon and plays a role in specifying this region [4] , [39] . It also has a role in development of the anterior placodes [13] , [40] . Such Foxg expression is induced by Fgf8, and Foxg maintains Fgf8 expression [41] . However, in ascidian embryos, Foxg was expressed only in the ANB and not in the brain, and Fgf8 is not expressed in the anterior part of the brain [38] . Consistently, we did not observe any obvious effects on the patterning and morphology of the brain in Foxg morphant embryos. These results strongly indicate that ascidian Foxg functions only in the ANB. In embryos of amphioxus, which was diverged before the split of ascidians and vertebrates, Foxg expression is found in a small region of the cerebral vesicle that is not considered to be the direct counterpart of the telencephalon [42] , although it is found in the nervous system after metamorphosis [43] . The expression patterns of Foxg in embryos of ascidians and amphioxus suggest that Foxg expression in the anterior brain was acquired in the vertebrate lineage after the split between these basal chordates and vertebrates. Foxg is expressed in the anterior ectoderm of a hemichordate embryo [44] . Because treatment with an FGF receptor inhibitor results in loss of Foxg expression in this animal [44] , Foxg might have been regulated by the MAPK signaling pathway before the emergence of chordates. We have previously demonstrated that transcriptional repressors Hes.a and Prdm1-r.a/b delay the onset of the specification program of the brain, and that this delay enables Foxc to be expressed in the ANB [8] , [45] . If this is indeed involved in emergence of the ANB in the common ancestor of ascidians and vertebrates, Foxg may subsequently be recruited as a downstream factor of Foxc as a specifier for the ANB. Then, Fgf8 might be recruited as a downstream factor of Foxg only in the vertebrate lineage. This recruitment would have constituted a mutual regulatory circuit, because Foxg had already been regulated by the MAPK pathway. A recent study proposed a model that incorporation of non-neural ectoderm was important for emergence of the vertebrate telencephalon [46] . Our data might extend this model; recruitment of Fgf8 might have strengthened Foxg expression in non-neural ectoderm. Alternatively, this recruitment may have induced Foxg in the brain region, because Fgf8 is a secreted signaling molecule. In other words, this circuit consisting of a transcription factor and signaling molecule might have enabled the Foxg expression domain to expand to the brain region of the vertebrate lineage. Animals and genes identifiers C. intestinalis (type A; also called C. robusta ) adults were obtained from the National Bio-Resource Project for Ciona intestinalis . This animal is excluded from legislation regulating scientific research on animals in Japan. Although there is no scientific evidence that Ciona can experience pain, discomfort or stress, we made our best efforts to minimize potential harm that Ciona individuals might experience when we obtained eggs and sperm from them. cDNA clones were obtained from our EST clone collection [47] . Identifiers [48] , [49] for genes examined in the present study were as follows: CG.KH2012.L57.25 for Foxc , CG.KH2012.C8.774 for Foxg , CG.KH2012.C3.553 for Six1/2 , CG.KH2012.L142.14 for Emx , CG.KH2012.L152.2 for Isl , CG.KH2012.C13.22 for Zf220 , CG.KH2012.L153.79 for Pitx , CG.KH2012.C4.341 for Foxb , CG.KH2012.C7.43 for Tfap2-r.b , CG.KH2012.C3.716 for Efna.d , CG.KH2012.C7.568 for Eph.c , and CG.KH2012.C10.174 for Meis . Gene knockdown and overexpression assays MOs (Gene Tools, LLC) against Foxg, Zf220 , Foxc , and Tfap2-r.b were used for the knockdown experiments [ Foxg (splicing block), 5′-AGTGCTGAACTTATAATCTACCTGT-3′; Foxg (translation block), 5′-GCGTCGTTCGTCATATTCTGTATGC-3′; Zf220 , 5′-ATAAAGACGACGTTTGAGCACTCAT-3′; Foxc , 5′-CATTGTCATTATAGAGAATCAAACC-3′, and Tfap2-r.b , 5′-CGGACAGAATTCGAATATCACTCAT-3′]. An MO against E. coli lacZ was used as the control (5′-TACGCTTCTTCTTTGGAGCAGTCAT-3′). The MOs against genes other than Foxg and Zf220 have been used previously and block translation [19] , [28] . We did not performed experiments to further confirm the specificity of these previously used MOs. The MOs were introduced by microinjection under a microscope. To confirm that the MO designed to block splicing of Foxg mRNA acted properly, we performed RT-PCR. 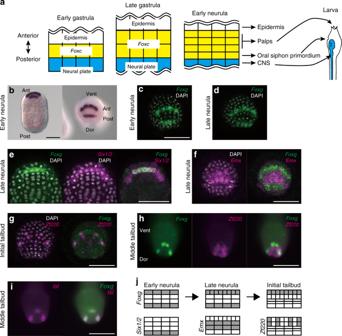Fig. 1 Foxgis specifically expressed in two rows of the anterior border of the neural plate.aSchematic illustrations of the anterior border of the neural plate in ascidian embryos. Epidermal cells, neural plate cells, and the intervening cells are represented by white, cyan, and yellow rectangles, respectively.b–dFoxgexpression revealed by chromatic and fluorescence in situ hybridization at the early and late neurula stages.Foxgis initially expressed in two separate rows during the neurula stage, and cells in the anterior row divide along the mediolateral axis until the late neurula stage.e–iDouble fluorescence in situ hybridization showing expression ofeFoxg(green) andSix1/2(magenta),fFoxg(green) andEmx(magenta),g,hFoxg(green) andZf220(magenta), andiFoxg(green) andIsl(magenta) at the late neurula to middle tailbud stages. Photographs are Z-projected image stacks overlaid in pseudocolor. The brightness and contrast of these photographs were adjusted linearly. Nuclei stained by DAPI are shown in gray in some photographs.jDepictions of the expression patterns ofFoxg, Six1/2,Emx, andZf220in the neural plate border at the neurula stage.b,eDorsal views in which the anterior is up.c,d,f–iAnterior views in which the ventral side is up. Ant anterior, Post posterior, Dor dorsal, Vent ventral. Scale bars represent 50 μm Primer sequences for Foxg were shown in Supplementary Table 1 . U0126 (Calbiochem, 662005) was used at 4 μM. The upstream sequence of Foxc (KHL57:96,056–98,200) was used for over/misexpression. Genes to be over/misexpressed were fused to the upstream sequence and introduced into fertilized eggs by electroporation. To prepare a dominant negative form of Eph.c, we cloned the region encoding the N-terminal 614 amino acid residues, which contained the extracellular domain and transmembrane domain, downstream to the Foxc upstream region. Gfp and Rfp genes were similarly fused to the same upstream or the upstream region of Foxg (KHC8:2,880,652–2,883,924), and used to mark the ANB and the anterior and posterior rows of the ANB. These constructs were introduced by electroporation unless noted otherwise. All knockdown and over/misexpression phenotypes were confirmed in at least two independent experiments. In situ hybridization and immunostaining For whole-mount in situ hybridization, digoxigenin (DIG)-RNA probes were synthesized by in vitro transcription with T7 RNA polymerase. Embryos were fixed in 4% paraformaldehyde in 0.1 M MOPS-NaOH (pH 7.5) and 0.5 M NaCl at 4 °C for overnight and then stored in 80% ethanol. After phosphate-buffered saline containing 0.1% tween 20 (PBST) wash, embryos were treated with 2 μg ml −1 Protenase K for 30 min at 37 °C, washed again with PBST, and fixed with 4% paraformaldehyde for 1 h at room temperature. Embryos were then incubated in 6x saline sodium citrate buffer (SSC), 50% formamide, 5x Denhardt’s solution, 100 μg mL −1 yeast tRNA, and 0.1% tween 20 for 1 h at 50 °C. After this prehybridization step, specific RNA probes were added and incubated for 48 h at 50 °C. Embryos were treated with RNase A, and incubated in 0.5x SSC, 50% formamide, and 0.1% tween 20 for 15 min at 50 °C twice. Embryos were further incubated in 0.5% blocking reagent (Roche) in PBST for 30 min, and then in 1:2000 alkaline-phosphatase-conjugated anti-DIG antibody (Roche). For chromogenic detection, embryos were further washed with 0.1 M NaCl, 50 mM MgCl 2 , and 0.1 M Tris-HCl (pH 9.5), and then NBT and BCIP were used for detection. For fluorescent detection, we used the TSA plus system (Perkin Elmer). To detect activation of the receptor-tyrosine kinase cascade, embryos were fixed with 3.7% formaldehyde, and treated with 3% H 2 O 2 for 30 min to quench endogenous peroxidase activity, and then incubated overnight with an anti-dpERK antibody (1:1000, Sigma, M9692) in Can-Get-Signal-Immunostain Solution B (TOYOBO). The signal was visualized with a TSA Kit (Invitrogen) using HRP-conjugated goat anti-mouse IgG and Alexa Fluor 488 tyramide. Gfp protein was similarly detected with an antibody against GFP (1:300, Thermo-Fisher Scientific, A6455). To visualize cell morphology, F-actin was stained with Alexa Fluor 555-conjugated phalloidin (Invitrogen). RT-PCR From neurula embryos, tailbud embryos, juveniles, and adults, RNA was extracted using the RNeasy mini kit (Qiagen), and reverse-transcribed with the oligo(dT) primer and Superscript III (Thermo Fisher Scientific). For pieces of juveniles, we used the Cell-to-Ct kit (Thermo Fisher Scientific) for RNA extraction and reverse-transcription. PCR was performed with GoTaq DNA polymerase (Promega). Ef1α was used for normalization. Primer sequences for Foxg and Ef1α were shown in Supplementary Table 1 . The used primers for Foxg were the same ones that we used for confirming that the Foxg MO acted properly. 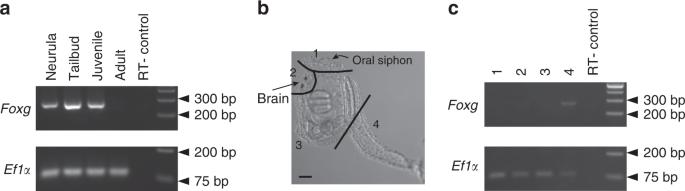Fig. 2 Foxgis not expressed in the nervous system after metamorphosis.aRT-PCR assay forFoxgexpression in neurula embryos, tailbud embryos, juveniles, and adults.Ef1αexpression was examined for a positive control. No amplification is observed in the negative control (RT- control), in which water was added instead of reverse transcriptase.bA juvenile in the same age used for RT-PCR in (a) and (c). For preparation of specimens used in (c), we cut animals into four pieces as indicated by lines. These four pieces are called specimens 1 to 4. The scale bar represents 50 μm.cRT-PCR assay forFoxgexpression in four pieces of juveniles.Ef1αexpression was examined for a positive control. NoFoxgexpression was detected in specimens 1 to 3 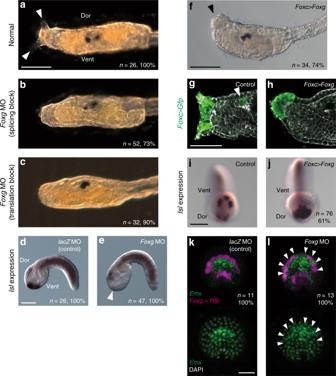Fig. 3 Foxgis essential for palp formation.a–cMorphology of the larval trunk developed fromacontrol unperturbed eggs,beggs injected with a MO designed to block splicing ofFoxgRNA, andceggs injected with a MO designed to block translation ofFoxgmRNA. While two of three palp protrusions are visible in normal embryos shown in (a) (arrowheads), no palp protrusions are visible in the morphants shown in (b) and (c).d,eIslexpression in embryos injected withdthe controllacZmRNA andetheFoxgMO. The palp-forming region lostIslexpression in theFoxgmorphant shown in (e) (arrowhead). Lateral views are shown.fA larva in whichFoxgwas over/misexpressed using the upstream region ofFoxcdeveloped a single large palp (arrowhead).g,hThe ANB cells were marked with GFP by introducing theFoxc>Foxgconstruct and counterstained with phalloidin (gray). The anterior trunk regions ofga control larva andha larva in whichFoxgwas over/misexpressed are shown.gIn normal embryos, ANB cells contribute to the palp region and the oral siphon primordium (arrowhead).hIn embryos withFoxgover/misexpression, all Gfp-positive cells were found in the single large palp.i,jIslexpression in (i) a control embryo and (j) an embryo withFoxgover/misexpression.Islis expressed in the entire palp-forming region in (j).k,lFluorescence in situ hybridization forEmxandRfp. Embryos were injected withkthelacZMO orltheFoxgMO.Foxg>Rfpwas coinjected to mark the most anterior and posterior rows of the ANB and detected by in situ hybridization. In (l), ectopic expression ofEmxwas detected in the anterior row. The number of embryos examined and the proportion of embryos that each panel represents are shown within the panels. The brightness and contrast of fluorescence images were adjusted linearly. Scale bars represent 50 μm 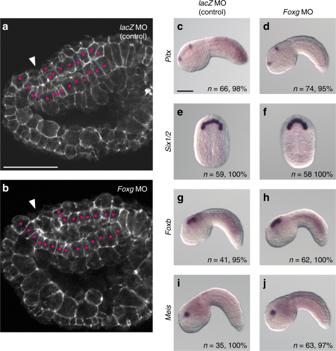Fig. 4 Knockdown ofFoxgdoes not affect the anterior part of the brain.a,bConfocal images of the trunk region of middle tailbud embryos injected withathelacZMO orbtheFoxgMO, which were stained with phalloidin. Arrowheads indicate the oral opening. Two layers of cells from the oral opening to the middle part of the brain are marked with magenta dots.c–jIn situ hybridization ofc,dPitx,e,fSix1/2,g,hFoxb, andi,jMeisin embryos injected withc,e,g,ithelacZMO ord,f,h,jtheFoxgMO. The number of embryos examined and the proportion of embryos that each panel represents are shown within the panels. Scale bars represent 50 μm 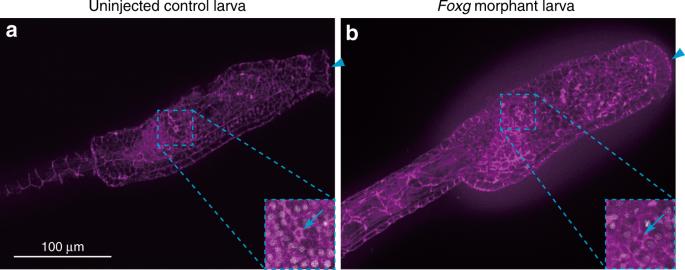Fig. 5 Knockdown ofFoxgdoes not affect the atrial siphon primordia. Z-projected images of the trunk region ofaa control larva andba larva developed from an egg injected with theFoxgMO, which were stained with phalloidin. Arrowheads indicates the anterior tip. Note that the palps were lost in theFoxgmorphant larva. Atrial siphon primordia in the right side are shown in higher magnification views. The openings are indicated by arrows. In higher magnification views, nuclei are stained by DAPI are shown in gray 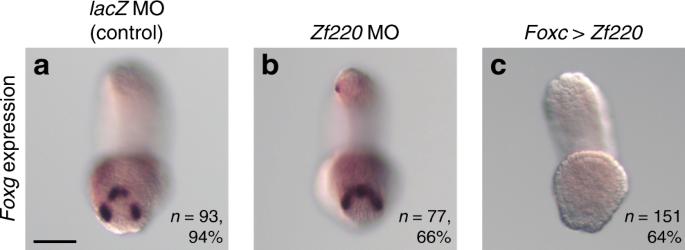Fig. 6 Zf220restrictsFoxgexpression to cells forming palp protrusions. In situ hybridization ofFoxgin tailbud embryos introduced withathelacZMO,btheZf220MO, andcan over/mis-expression construct ofZf220(Foxc>Zf220). The number of embryos examined and the proportion of embryos that each panel represents are shown within the panels. The scale bar in (a) represents 50 μm 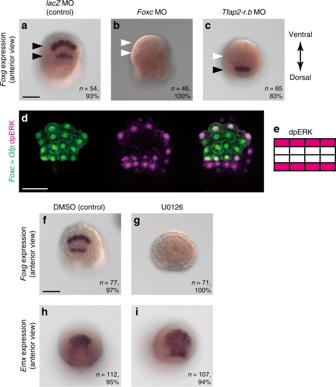Fig. 7 Upstream mechanism that regulates specific expression ofFoxg.a–cFoxgexpression in embryos injected withathelacZcontrol MO,btheFoxcMO, andctheTfap2-r.bMO. Rows that expressFoxgare shown by black arrowheads, and rows that lose the expression are shown by white arrowheads.dImmunostaining of dpERK (magenta) in an embryo in which ANB cells were marked withFoxc>Gfp. The brightness and contrast of fluorescence images were adjusted linearly. Note that dpERK signals are also seen in the most anterior row of the neural plate.eDepiction of dpERK-positive cells in the ANB.f–iIn situ hybridization off,gFoxgandh,iEmxinf,hcontrol embryos andg,iembryos treated with U0126. The number of embryos examined and the proportion of embryos that each panel represents are shown within the panels. The scale bar in (a) represents 50 μm 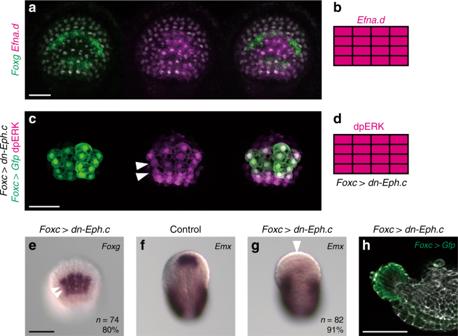Fig. 8 Efna.dis responsible for restrictingFoxgexpression in the ANB.aDouble in situ hybridization ofEfna.d(magenta) andFoxg(green).bDepiction forEfna.dexpression in the ANB.cImmunostaining of dpERK (magenta) in an embryo in which ANB cells were marked withFoxc>Gfp. The middle rows show ectopic signals for dpERK (arrowheads).dDepiction of ANB cells stained with the anti-dpERK antibody in neurula embryos introduced withFoxc>dn-Eph.c.e–gIn situ hybridization ofeFoxgandf,gEmxine,gneurula embryos introduced withFoxc>dn-Eph.candfan unperturbed neurula embryo. In (e), the middle two rows of cells expressedFoxgectopically (compared with Fig.1b). In (f) and (g), whileEmxexpression in the tail was not changed, it was lost in the ANB of aFoxgmorphant (arrowhead). The number of embryos examined and the proportion of embryos that each panel represents are shown within the panels.a,c,eAnterior views in which the ventral side is up.f,gDorsal views in which the anterior is up.hLateral view showing the morphology of a larva introduced withFoxc>dn-Eph.c. ANB cells were marked with GFP by cointroduction of theFoxc>Gfpconstruct and counterstained with phalloidin (gray) 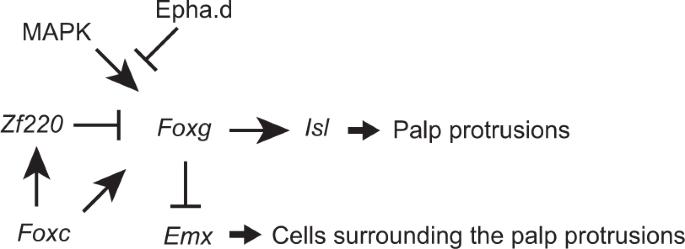Fig. 9 Foxgplays a central role in patterning the ANB. The gene regulatory circuit in the ANB revealed by the present and previous studies7,12,18,19 Reporting summary Further information on research design is available in the Nature Research Reporting Summary linked to this article.